Inflammation-induced proteolytic processing of the SIRPα cytoplasmic ITIM in neutrophils propagates a proinflammatory state Signal regulatory protein α (SIRPα), an immunoreceptor tyrosine-based inhibitory motif (ITIM)-containing receptor, is an essential negative regulator of leukocyte inflammatory responses. Here we report that SIRPα cytoplasmic signalling ITIMs in neutrophils are cleaved during active inflammation and that the loss of SIRPα ITIMs enhances the polymorphonuclear leukocyte (PMN) inflammatory response. Using human leukocytes and two inflammatory models in mice, we show that the cleavage of SIRPα ITIMs in PMNs but not monocytes occurs at the post-acute stage of inflammation and correlates with increased PMN recruitment to inflammatory loci. Enhanced transmigration of PMNs and PMN-associated tissue damage are confirmed in mutant mice expressing SIRPα but lacking the ITIMs. Moreover, the loss of SIRPα ITIMs in PMNs during colitis is blocked by an anti-interleukin-17 (IL-17) antibody. These results demonstrate a SIRPα-based mechanism that dynamically regulates PMN inflammatory responses by generating a CD47-binding but non-signalling SIRPα ‘decoy’. Serving as the first line of defence against pathogen invasion, the response of neutrophils (polymorphonuclear leukocytes (PMNs)) is a central component of active inflammation. However, the infiltration of large numbers of PMNs into tissues is also the major cause of severe tissue damage, as observed in many inflammatory diseases. Although the precise mechanisms regulating PMN function during inflammation remain incompletely understood, previous studies by us and others demonstrate that signal regulatory protein α (SIRPα) and its interactions with CD47 have an important role [1] , [2] . SIRPα, a receptor-like cell surface signalling molecule that is predominantly expressed by myeloid leukocytes [3] , [4] , [5] , contains an extracellular domain that comprises two IgC-like loops and one IgV-like loop. The extracellular binding of SIRPα to CD47 occurs via the IgV loop [6] . In addition to a single transmembrane domain, SIRPα contains a cytoplasmic tail that bears two important signalling motifs that are often found in immune cells: immunoreceptor tyrosine-based inhibitory motifs (ITIMs). It has been shown that phosphorylation of the tyrosine residues in SIRPα ITIMs provides docking sites for the recruitment of Src homology 2 domain-containing protein tyrosine phosphatases (SHP-1 or SHP-2) [4] , [7] , [8] , which in turn triggers downstream signalling events that result in the negative regulation of cell function. In macrophages, SIRPα-mediated signalling controls the phagocytosis of self cells [9] , [10] . More specifically, the ligation of SIRPα on macrophages by CD47 expressed on tissue cells induces the phosphorylation of ITIMs and leads to the inhibition of macrophage phagocytosis, whereas the failure of SIRPα cell surface engagement or ITIM phosphorylation-mediated signalling promotes macrophage phagocytosis [4] . In PMNs and monocytes, it was shown that perturbation of SIRPα interactions by antibodies or a soluble CD47 extracellular domain impedes the chemotactic transmigration of these cells across endothelial or epithelial monolayers [1] , [2] . Compared with macrophages, in which the mechanisms of SIRPα’s effects have been studied to a certain extent, the regulation of SIRPα in PMNs has not been well studied. PMNs are heterogeneous and present various inflammatory statuses, probably as a result of priming by different chemoattractants or cytokines. Previous studies have shown upregulation of CD11b/CD18 (Mac-1) and CD66b, and downregulation of L-selectin in PMNs in response to various cytokines or chemotaxins [11] . The interpretation of these studies, however, is hampered by the fact that the primed and activated states of PMN cells remain poorly defined. It remains unknown whether SIRPα is altered during PMN priming and whether such alteration affects the role of SIRPα in regulating the PMN response during the dynamic course of inflammation. Here we report the first piece of evidence, indicating that active inflammation can induce the formation of an extracellular ligand-binding but signal-less SIRPα ‘decoy’ on the PMN cell surface through the specific cleavage of the SIRPα cytoplasmic ITIMs. We further demonstrate that PMNs bearing ITIM-free SIRPα display an enhanced proinflammatory phenotype. Our results describe a novel mechanism underlying the dynamic interplay between leukocytes and inflammation, and show that chronic inflammation induces reprogramming of PMN response. Heterogeneous SIRPα in PMNs To study SIRPα expression in PMNs and monocytes, human PMNs and peripheral blood mononuclear cells (PBMCs) were freshly isolated from healthy volunteers and tested using SIRPα extracellular domain (anti-SIRPα.ex), an antibody that specifically recognizes the extracellular domain of SIRPα. To minimize cross-reactivity with SIRPβ [6] , this antibody was immuno-absorbed by an immobilized recombinant SIRPβ extracellular domain before use. As shown in Fig. 1a , anti-SIRPα.ex detected SIRPα in PMNs and monocytes (PBMCs) as a glycoprotein with a molecular weight (MW) of <85 kDa. This protein was further confirmed to be SIRPα by pull down assay, with a soluble CD47 extracellular domain, CD47-AP [12] , which bound to SIRPα but not to SIRPβ. It was also confirmed that the anti-SIRPα.ex antibody has minimal cross-reactivity with SIRPβ, which presented as a homodimer with an MW of 110 kDa under non-reducing conditions [12] ( Supplementary Figure S1 ). Although it was detected in both cell types, SIRPα displayed a much broader MW range (65–85 kDa) in PMNs than in monocytes (75–85 kDa; Fig. 1a ). We also blotted the same PMN and PBMC lysates using another specific anti-SIRPα antibody, anti-SIRPα.ct, which detects the cytoplasmic carboxy terminus ( Fig. 1c ). Interestingly, anti-SIRPα.ct consistently detected SIRPα in PBMCs but occasionally reacted poorly with PMNs or detected a pattern that was different from the pattern observed when using anti-SIRPα.ex ( Fig. 1a ). To understand the differences in SIRPα between PMNs and monocytes, we performed protein deglycosylation using PNGase F. As shown in Fig. 1b , SIRPα in monocytes was decreased to 55 kDa after deglycosylation, which corresponds to the expected core size of 503/504 amino acids. However, SIRPα in PMNs was resolved as three deglycosylated bands: 55, 50 and 45 kDa. 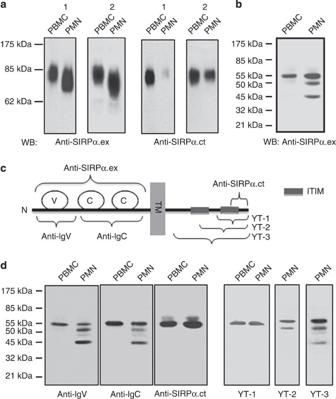Figure 1: Differential expression of SIRPα in PMNs and PBMCs. (a) Detection of SIRPα in human PMNs and PBMCs by WB analysis. Freshly isolated human PMNs and PBMCs were lysed and subjected to SDS–PAGE under non-reducing conditions, followed by immunoblotting using antibodies against the extracellular domain (anti-SIRPα.ex) and the C-terminus of the intracellular domain (anti-SIRPα.ct). The figure shows the WB results of PMN and PBMCs obtained from two randomly selected donors (1 and 2). (b) Protein deglycosylation of human PMN and PBMC lysates by PNGase F followed by WB using anti-SIRPα.ex revealed multiple forms of SIRPα in PMNs. (c) Schematic illustration of the epitope regions of SIRPα recognized by the different anti-SIRPα antibodies. The SIRPα protein is shown to contain one IgV-like (V) loop and two IgC-like (C) loops in the extracellular domain. TM, transmembrane domain; ITIM, immunotyrosine-based inhibitory motif; YT-1, 2, 3 are the polyclonal antibodies generated against different regions of SIRPα cytoplasmic tail. (d) WB of deglycosylated PMN and PBMC lysates using different anti-SIRPα antibodies. Figure 1: Differential expression of SIRPα in PMNs and PBMCs. ( a ) Detection of SIRPα in human PMNs and PBMCs by WB analysis. Freshly isolated human PMNs and PBMCs were lysed and subjected to SDS–PAGE under non-reducing conditions, followed by immunoblotting using antibodies against the extracellular domain (anti-SIRPα.ex) and the C-terminus of the intracellular domain (anti-SIRPα.ct). The figure shows the WB results of PMN and PBMCs obtained from two randomly selected donors (1 and 2). ( b ) Protein deglycosylation of human PMN and PBMC lysates by PNGase F followed by WB using anti-SIRPα.ex revealed multiple forms of SIRPα in PMNs. ( c ) Schematic illustration of the epitope regions of SIRPα recognized by the different anti-SIRPα antibodies. The SIRPα protein is shown to contain one IgV-like (V) loop and two IgC-like (C) loops in the extracellular domain. TM, transmembrane domain; ITIM, immunotyrosine-based inhibitory motif; YT-1, 2, 3 are the polyclonal antibodies generated against different regions of SIRPα cytoplasmic tail. ( d ) WB of deglycosylated PMN and PBMC lysates using different anti-SIRPα antibodies. Full size image To characterize the three SIRPα species in PMNs, we generated additional antibodies, designated YT-1, YT-2 and YT-3, against various cytoplasmic regions of SIRPα and two polyclonal antibodies, anti-IgV and anti-IgC, which recognize the extracellular IgV and IgC loops, respectively ( Fig. 1c ). YT-3 was generated using the entire intracellular domain of SIRPα as the antigen, whereas YT-1 and YT-2 were produced using C-terminal peptides that covered either one or two ITIMs, respectively. As shown in Fig. 1d , both anti-IgV and anti-IgC detected an identical pattern of three SIRPα bands in PMNs, suggesting that all of these SIRPα species share a similar extracellular structure. Among four antibodies against the cytoplasmic domain, YT-3 recognized all three SIRPα species, whereas YT-1, YT-2 and anti-SIRPα.ct detected only the 55-kDa band. As these three antibodies detect the ITIMs-containing tail, these results suggest that only the 55-kDa SIRPα, and not the two smaller species, contain ITIMs. Thus, in contrast to monocytes, which express only intact SIRPα, PMNs contain heterogeneous SIRPα proteins. In addition to the intact ITIM-containing ‘signalling’ SIRPα (designated as ITIM + SIRPα), PMNs also produce a non-signalling ITIM-less SIRPα (designated as ITIM − SIRPα). Loss of SIRPα ITIMs in PMNs is associated with inflammation To determine whether different SIRPα expression in PMNs is due to donor variation, we isolated leukocytes from more than 30 randomly selected, self-declared healthy donors, and examined SIRPα expression in all samples. As shown in Fig. 2a , SIRPα in most of the PMN samples (70–80%) and in all monocyte samples (100%) was recognized by both the anti-SIRPα.ex and the anti-SIRPα.ct antibodies. However, ~ 20–30% of the PMN samples (marked by ‘*’) showed diminished recognition by anti-SIRPα.ct, suggesting a likelihood of reduction in ITIM + SIRPα expression and of primary expression of ITIM − SIRPα. This interesting result prompted us to examine whether the presence or absence of ITIM + SIRPα in PMNs reflected different phenotypes of these cells and whether these differences affect PMN function. As PMNs are highly sensitive to and can be primed by inflammatory factors, we hypothesized that the donors whose PMNs lacked ITIM + SIRPα might experience mild inflammation without noticeable effects. To test this possibility, we obtained PMNs from one donor with active gout (inflammatory arthritis), one donor with upper respiratory allergies and two donors with throat and/or upper respiratory inflammation following a typical cold. As shown in Fig. 2b , all of the PMN samples displayed a marked decrease in or complete loss of SIRPα recognition by the anti-SIRPα.ct antibody. Protein deglycosylation ( Fig. 2b , lower panel) confirmed that these PMNs lacked the 55-kDa ITIM + SIRPα and contained only the smaller ITIM − SIRPα. Decreased recognition by the anti-SIRPα.ct antibody in these PMNs was not due to the downregulation of total SIRPα, as anti-SIRPα.ex reacted in a manner similar to that of controls ( Fig. 2b ). As expected, later re-examination of PMNs from the same donors, after these individuals had recovered from the cold or allergies, or after the acute gout subsided, found increases in ITIM + SIRPα to levels similar to those of most healthy donors ( Fig. 2c ). We also detected SIRPβ using a SIRPβ-specific antibody (clone B4B6) [13] and found no noticeable alteration in the PMNs from all donors ( Fig. 2c ). As the alteration of SIRPα occurred only in the intracellular tail, we tested SIRPα binding to CD47 via the extracellular domain. For this purpose, PMN lysates were immobilized, and binding to CD47-AP [14] was assayed by dot blots. As shown in Supplementary Fig. S2A , no alteration of CD47-AP binding to various PMN lysates was observed. Together, these results suggest that PMNs in healthy donors generally contain ITIM + SIRPα, whereas inflammatory conditions induce the formation of ITIM-less SIRPα. In addition, this change in SIRPα is PMN-specific, as monocytes obtained from the same donors consistently expressed only ITIM + SIRPα ( Fig. 2a ). 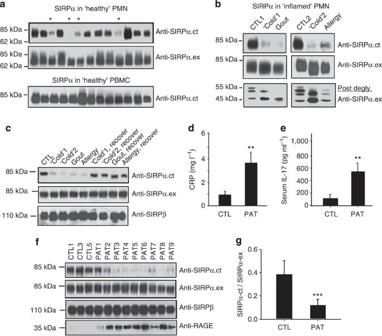Figure 2: The correlation between the loss of SIRPα ITIMs in PMN and active inflammation. (a) Peripheral PMNs and PBMCs were isolated from randomly selected ‘healthy’ donors. WB analyses of SIRPα expression by anti-SIRPα.ex and anti-SIRPα.ct antibodies. The samples that had decreased reactivity with anti-SIRPα.ct are marked ‘*’. (b) PMNs obtained from a donor with active gout, two donors with upper respiratory inflammation (‘Cold’) and a donor with upper respiratory allergies were analysed for SIRPα protein. PMNs from two healthy donors were used as controls (CTL1 and CTL2). Protein deglycosylation results were shown in the lower panel. (c) Recovery of anti-SIRPα.ct reactivity in PMNs isolated from the same donors after their ‘cold’, gout or allergy was subsided. (d) Levels of C-reactive protein (CRP) and (e) levels of IL-17 in plasma of healthy donors (CTL,n=12) and type 2 diabetic patients with cardiovascular complications (PAT,n=25) detected by enzyme-linked immunosorbent assay. The data presented as means±s.d., **P<0.01 determined by Student’st-test. (f,g) WB analyses of SIRPα in PMNs of 25 type 2 diabetic patients with cardiovascular complications (PAT) and 12 healthy controls (CTL). RAGE, receptor for advanced glycation end products. Note that the WB images (f) show partial results, whereas the densitometry analysed all PMN samples (g). The data presented as means±s.d., ***P<0.005 determined by Student’st-test. Figure 2: The correlation between the loss of SIRPα ITIMs in PMN and active inflammation. ( a ) Peripheral PMNs and PBMCs were isolated from randomly selected ‘healthy’ donors. WB analyses of SIRPα expression by anti-SIRPα.ex and anti-SIRPα.ct antibodies. The samples that had decreased reactivity with anti-SIRPα.ct are marked ‘*’. ( b ) PMNs obtained from a donor with active gout, two donors with upper respiratory inflammation (‘Cold’) and a donor with upper respiratory allergies were analysed for SIRPα protein. PMNs from two healthy donors were used as controls (CTL1 and CTL2). Protein deglycosylation results were shown in the lower panel. ( c ) Recovery of anti-SIRPα.ct reactivity in PMNs isolated from the same donors after their ‘cold’, gout or allergy was subsided. ( d ) Levels of C-reactive protein (CRP) and ( e ) levels of IL-17 in plasma of healthy donors (CTL, n =12) and type 2 diabetic patients with cardiovascular complications (PAT, n =25) detected by enzyme-linked immunosorbent assay. The data presented as means±s.d., ** P <0.01 determined by Student’s t -test. ( f , g ) WB analyses of SIRPα in PMNs of 25 type 2 diabetic patients with cardiovascular complications (PAT) and 12 healthy controls (CTL). RAGE, receptor for advanced glycation end products. Note that the WB images ( f ) show partial results, whereas the densitometry analysed all PMN samples ( g ). The data presented as means±s.d., *** P <0.005 determined by Student’s t -test. Full size image To confirm that the loss of ITIM + SIRPα in PMNs is associated with inflammation, we further tested PMNs obtained from 25 donors who had type 2 diabetes complicated by coronary dysfunction. In addition, 12 healthy donors (CTL) were enroled in the study. As shown in Fig. 2f , all diabetic individuals (PAT) manifested decreased or diminished recognition by the anti-SIRPα.ct antibody, whereas recognition by the anti-SIRPα.ex antibody or anti-SIRPβ antibody (monoclonal antibody B4B6) remained the same as in the controls. Despite the depletion of ITIMs, dot blot analyses indicated that the SIRPα extracellular domains in diabetic PMNs were functional and directly bound to CD47-AP ( Supplementary Fig. S2B ). In addition, we detected elevations in C-reactive protein and interleukin (IL)-17 in the plasma [15] ( Fig. 2d,e ) and increased expression of receptor for advanced glycation end products ( Fig. 2f ), a diabetes-associated inflammation propagator [16] , in diabetic PMNs. The elevation of receptor for advanced glycation end products in the patients confirmed their diabetic condition in conjunction with active inflammation [17] . Studies using mouse inflammation models Two murine inflammation models, dextran sulphate sodium (DSS)-induced colitis [18] and streptozotocin (STZ)-induced diabetes [19] , were used to study SIRPα alterations in PMNs during inflammation. In agreement with previous reports, 2% DSS treatment caused progressive colitis, resulting in significant body weight loss, PMN infiltration into the intestines and mucosal damage ( Supplementary Fig. S3 ). Examination of SIRPα in PMNs, as shown in Fig. 3 , using an antibody against the mouse-specific SIRPα extracellular domain (monoclonal antibody P84) indicated consistent SIRPα expression. However, simultaneous detection using anti-SIRPα.ct revealed diminishment of the cytoplasmic tail starting at approximately day 6 of the DSS treatment, which was suggestive of ITIM + SIRPα depletion during inflammation progression. Interestingly, the time course of ITIM + SIRPα loss matched significant elevation in the proinflammatory cytokine IL-17 in the serum. As shown in Fig. 3c and in previous studies [20] , [21] , remarkable levels of IL-17 were induced after 6 days of DSS treatment during colitis development. This high level of IL-17 at the post-acute/chronic stage of colitis has a role in aggravation of the inflammatory condition. Moderate increases in IL-6 were also observed. 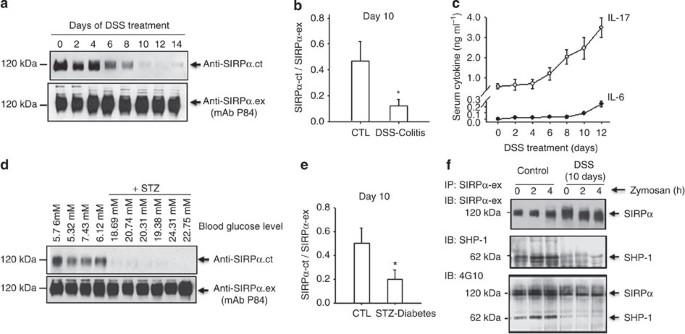Figure 3: Deletion of the SIRPα cytoplasmic ITIMs in mouse PMNs under inflammatory conditions. (a) WT mice were induced colitis by feeding with 2% DSS in the drinking water. At different days of the treatment, bone marrow PMNs were isolated from the mice and were analysed for SIRPα by WB using a murine-specific anti-SIRPα.ex (mAb P84) and anti-SIRPα.ct. (b) WB analyses of SIRPα in PMNs obtained from non-DSS-treated mice (CTL) and colitic mice that were treated with 2% DSS for 10 days. The reactivity of anti-SIRPα.ex (mAb P84) versus anti-SIRPα.ct was analysed by densitometry;n=5 mice per group. The data are presented as means±s.d., *P<0.05 determined by Student’st-test. (c) The serum levels of the proinflammatory cytokine IL-17 and IL-6 in DSS-treated mice. Note that the loss of SIRPα cytoplasmic ITIMs in PMNs correlated with the high elevation of IL-17, both starting at approximately day 6 during the DSS treatment. (d) WT mice were induced diabetes by STZ administration. Two weeks after the hyperglycaemic conditions were stably established, bone marrow PMNs were analysed for SIRPα by WB. The data are presented as means±s.e.m. (e) Densitometry analyses of SIRPα WB analysis are shown ind. The data are presented as means±s.d., *P<0.05 determined by Student’st-test. The data are representative of one of five individual experiments. (g) Defects in the recruitment and phosphorylation of SHP-1 in PMN from DSS-treated C57BL/6J WT mice during zymosan–peritonitis. IP, immunoprecipitation; IB, immunoblot. Figure 3: Deletion of the SIRPα cytoplasmic ITIMs in mouse PMNs under inflammatory conditions. ( a ) WT mice were induced colitis by feeding with 2% DSS in the drinking water. At different days of the treatment, bone marrow PMNs were isolated from the mice and were analysed for SIRPα by WB using a murine-specific anti-SIRPα.ex (mAb P84) and anti-SIRPα.ct. ( b ) WB analyses of SIRPα in PMNs obtained from non-DSS-treated mice (CTL) and colitic mice that were treated with 2% DSS for 10 days. The reactivity of anti-SIRPα.ex (mAb P84) versus anti-SIRPα.ct was analysed by densitometry; n =5 mice per group. The data are presented as means±s.d., * P <0.05 determined by Student’s t -test. ( c ) The serum levels of the proinflammatory cytokine IL-17 and IL-6 in DSS-treated mice. Note that the loss of SIRPα cytoplasmic ITIMs in PMNs correlated with the high elevation of IL-17, both starting at approximately day 6 during the DSS treatment. ( d ) WT mice were induced diabetes by STZ administration. Two weeks after the hyperglycaemic conditions were stably established, bone marrow PMNs were analysed for SIRPα by WB. The data are presented as means±s.e.m. ( e ) Densitometry analyses of SIRPα WB analysis are shown in d . The data are presented as means±s.d., * P <0.05 determined by Student’s t -test. The data are representative of one of five individual experiments. ( g ) Defects in the recruitment and phosphorylation of SHP-1 in PMN from DSS-treated C57BL/6J WT mice during zymosan–peritonitis. IP, immunoprecipitation; IB, immunoblot. Full size image Similarly, a loss of ITIM + SIRPα in PMNs was observed in STZ-induced diabetic mice, as shown in Fig. 3d,e . The mice that were treated with STZ all developed hyperglycaemia (mean blood glucose levels: 26.9±5.1 mM for the STZ group versus 7.4±2.1 mM for the control group). Analyses of SIRPα in PMNs isolated from the hyperglycaemic mice again indicated decreases in ITIM + SIRPα, as detected by anti-SIRPα.ct. No decrease in total SIRPα in PMNs or in ITIM + SIRPα in monocytes or macrophages was observed in either the DSS- or the STZ-treated mice. Given that the SIRPα cytoplasmic ITIMs are essential for initiating negative signalling events by recruiting SHP-1/2 (refs 8 , 22 ), we analysed whether the loss of SIRPα ITIMs in PMNs under inflammatory conditions leads to defects in SHP binding. For these experiments, mice with or without treatment with DSS for 10 days received an intraperitoneal injection of zymosan A to induce peritonitis. At 2 and 4 h after the zymosan injection, PMNs were isolated from the bone marrow, and the phosphorylation of SIRPα and its coprecipitation with SHP-1 were examined. As shown in Fig. 3f , in PMNs from non-DSS-treated mice, phosphorylated SIRPα was co-immunoprecipitated with SHP-1, and the recruited SHP-1 was also phosphorylated. In contrast, the relative phosphorylation of SIRPα and its association with SHP-1 in PMNs from DSS-treated mice were diminished. Loss of SIRPα ITIMs promotes PMN infiltration Our previous studies demonstrated that PMN infiltration is significantly enhanced when inflammatory conditions proceed into the post-acute or chronic stage [20] . We determined whether the loss of ITIM + SIRPα correlates with enhanced PMN infiltration. Zymosan-induced peritonitis [20] was induced to assay PMN infiltration in vivo. As shown in Fig. 4a,b , in mice without an ongoing chronic condition, only few PMNs (<2.0 × 10 6 ) were detected in the peritoneum at 2 h after zymosan injection, whereas major PMN infiltration occurred at 4–6 h. In contrast, significantly accelerated PMN infiltration and, hence, greatly increased PMN accumulation in the peritoneum at 2 h, was detected in the mice treated with DSS for over 6 days, but not for a shorter period, and in mice with chronic hyperglycaemia (STZ). Analyses of the kinetic enhancement of PMN infiltration in DSS-treated mice found a tight correlation with the reduction in SIRPα cytoplasmic ITIMs in PMNs, as both events occurred after 6 days of DSS treatment. As shown in the previous figure, the marked elevation of serum IL-17 also occurred at the same time point ( Fig. 3c ). To test whether the elevation of IL-17 was causally related to the deletion of ITIMs in SIRPα and to enhanced PMN transmigration, mice were administered recombinant IL-17A (20 μg, intravenously [21] every other day for three times total. SIRPα was then analysed in PMNs. As shown in Fig. 4c,d , IL-17 treatment directly led to a depletion of ITIM + SIRPα in PMNs. In contrast, neutralization of IL-17 during DSS-induced colitis by an intravenous injection of an anti-IL-17 antibody [20] , [23] ( Fig. 4e ) prevented the deletion of SIRPα ITIMs ( Fig. 4f,g ) and eliminated the enhancement of PMN infiltration ( Fig. 4h ). These results thus suggest that elevated IL-17 during colitis promotes SIRPα alteration in PMNs, leading to an enhancement of PMN infiltration. 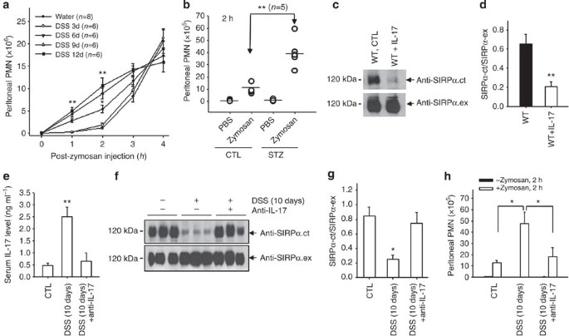Figure 4: PMN bearing ITIM–SIRPα have enhanced peritoneal infiltration and IL-17 promotes ITIM–SIRPα formation. (a) Control mice (water) and mice treated with DSS for various days were injected with 0.5 mg zymosan A followed by analyses of PMN infiltration into the peritoneum at different time points. (b) Mice with/without STZ treatment were injected with zymosan A followed by analysis of PMN migration into the peritoneum at 2 h. The results inaare presented as means±s.d., representing three to five independent experiments with multiple mice per group. *P<0.05; **P<0.01 as assessed by Student’st-test. (c,d) IL-17 treatment (20 μg IL-17A, intravenously every other day for a total of three times) resulted in the loss of SIRPα cytoplasmic ITIMs in mouse bone marrow PMN. The data are presented as means±s.d., **P<0.01 determined by Student’st-test. (e) Inhibition of IL-17 by the administration of an anti-mouse IL-17A antibody (50 μg, intravenously) on days 6 and 9 during DSS treatment. Anti-IL-17A antibody administration prevented the cleavage of SIRPα cytoplasmic ITIMs in PMNs (f,g) and abolished the enhancement of PMN infiltration during DSS treatment (h). The results are presented as means±s.d. and represent three independent experiments with three to five mice per condition. *P<0.05; **P<0.01 as assessed by Student’st-test. Figure 4: PMN bearing ITIM–SIRPα have enhanced peritoneal infiltration and IL-17 promotes ITIM–SIRPα formation. ( a ) Control mice (water) and mice treated with DSS for various days were injected with 0.5 mg zymosan A followed by analyses of PMN infiltration into the peritoneum at different time points. ( b ) Mice with/without STZ treatment were injected with zymosan A followed by analysis of PMN migration into the peritoneum at 2 h. The results in a are presented as means±s.d., representing three to five independent experiments with multiple mice per group. * P <0.05; ** P <0.01 as assessed by Student’s t -test. ( c , d ) IL-17 treatment (20 μg IL-17A, intravenously every other day for a total of three times) resulted in the loss of SIRPα cytoplasmic ITIMs in mouse bone marrow PMN. The data are presented as means±s.d., ** P <0.01 determined by Student’s t -test. ( e ) Inhibition of IL-17 by the administration of an anti-mouse IL-17A antibody (50 μg, intravenously) on days 6 and 9 during DSS treatment. Anti-IL-17A antibody administration prevented the cleavage of SIRPα cytoplasmic ITIMs in PMNs ( f , g ) and abolished the enhancement of PMN infiltration during DSS treatment ( h ). The results are presented as means±s.d. and represent three independent experiments with three to five mice per condition. * P <0.05; ** P <0.01 as assessed by Student’s t -test. Full size image To confirm that the loss of ITIM + SIRPα directly enhances the PMN inflammatory response, we employed genetically modified mice (designated as SIRPα.ct −/− in this study) in which most of the SIRPα cytoplasmic domain, including both ITIMs, was deleted [24] . SIRPα.ct −/− mice showed no noticeable differences in body weight and peripheral white blood cell count compared with their wild-type (WT) littermates [25] . Assaying PMN infiltration by zymosan-induced peritonitis indicated greater (~ 20%) in PMN recruitment into the peritoneum at early time points (2–3 h) in homozygous SIRPα.ct −/− mice than in heterozygous (SIRPα.ct +/− ) or WT littermates ( Fig. 5a,b ). Inducing colitis by 2% DSS also revealed that SIRPα.ct −/− mice developed much more severe colitis than their WT littermates. As shown in Fig. 5c,d , SIRPα.ct −/− mice demonstrated more rapid body weight loss and quickly succumbed to the condition in a few days. More severe mucosal epithelial damage associated with enhanced PMN infiltration in SIRPα.ct −/− mice relative to WT controls was also observed ( Supplementary Fig. S3 ). In-vitro assays of PMN chemotaxis and PMN production of reactive oxygen species upon challenge also demonstrated that PMNs bearing ITIM − SIRPα derived from SIRPα.ct −/− mice had enhanced responses compared with PMNs with ITIM + SIRPα from WT littermates ( Fig. 5e,f ). Co-adoptive transfer experiments were performed to further examine the association of the ITIM deletion in SIRPα with enhanced PMN recruitment during inflammation. As depicted in Fig. 5g , PMNs isolated from the bone marrow of SIRPα.ct −/− mice and their WT littermates (SIRPα.ct +/+ ) were labelled with the cellular dyes carboxyfluorescein succinimidyl ester (CFSE, green) and 7-hydroxy-9H-(1,3-dichloro-9,9-dimethylacridin-2-one)-succinimidyl ester (DDAO-SE, CellTrace Far Red). Equal amounts of CFSE-labelled and DDAO-SE-labelled PMNs were then intravenously injected into the same WT mice in which peritonitis has been induced by zymosan. As shown in Fig. 5h,i , there were more SIRPα.ct −/− PMNs recovered from the peritoneum than SIRPα.ct +/+ PMNs at the early stage of peritonitis. 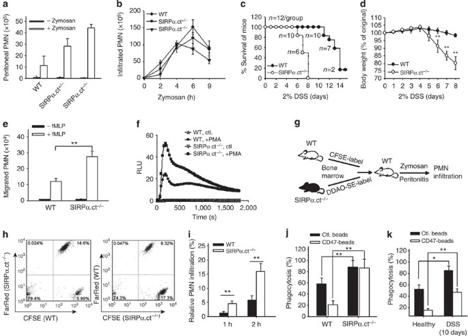Figure 5: Genetic deletion of SIRPα ITIMs augments PMN migration towards inflammatory loci. (a)In-vivoassay of PMN infiltration. WT mice and mice bearing the SIRPα cytoplasmic domain deletion (homozygous SIRPα.ct−/−and heterozygous SIRPα.ct+/−) were intraperitoneally injected with zymosan, and PMN recruitment into the peritoneum at 2 h was assayed. (b) Time-course analyses of PMN accumulation at the peritoneum during zymosan-induced peritonitis. In addition to peritonitis, mice were induced colitis by 2% DSS. The SIRPα.ct−/−mice were characterized as having more severe DSS-induced colitis than their WT littermates, as determined by their lower survival rate (c) and more rapid weight loss (d). The data ina,banddare presented as means±s.d., withn=6 in each condition. (e)In-vitrochemotaxis assay. PMN (2.5 × 106) obtained from SIRPα.ct−/−mice and WT littermates were induced by 10 μM fMLP to migrate across collagen-coated transwell filters. Transmigrated PMNs over a 1-h period were measured by an myeloperoxidase assay. The data are presented as means±s.d. and represent five independent experiments with triplicates per condition. (f) Reactive oxygen species production upon PMA challenge. PMN (5 × 105) from SIRPα.ct−/−mice and WT littermates were loaded with 200 μM luminol (Sigma). Following stimulation with PMA (1 μM), chemiluminescence was measured at 37 °C in relative light units (RLU) at every 30 s over a period of 30 min. (g) Illustration of co-adoptive transfer of PMNs from SIRPα.ct−/−and WT littermates followed by assay PMN infiltration during zymosan-induced peritonitis. (h) Infiltration of SIRPα.ct−/−PMN and SIRPα.ct+/+PMN in the same WT mice at 2 h during zymosan–peritonitis. Note that SIRPα.ct−/−and WT PMNs were cross-labelled with either CFSE or DDAO-SE before transfer into the recipient mice. Fluorescence-activated cell sorting analyses of PMNs at 1 and 2 h (i) during peritonitis revealed more SIRPα.ct−/−PMN than WT PMN. (j) PMN phagocytosis of fluorescent beads coated with/without CD47 extracellular domain. SIRPα.ct−/−and WT PMNs were collected from the peritoneum during peritonitis at 3 h. (k) WT mice treated with water or DSS for 10 days were induced peritonitis by zymosan. PMNs collected from the peritoneum at 3 h were tested for phagocytosis. The results (i,jandk) are presented as means±s.d. with triplicates in each condition. *P<0.05; **P<0.01 as assessed by Student’st-test. Figure 5: Genetic deletion of SIRPα ITIMs augments PMN migration towards inflammatory loci. ( a ) In-vivo assay of PMN infiltration. WT mice and mice bearing the SIRPα cytoplasmic domain deletion (homozygous SIRPα.ct −/− and heterozygous SIRPα.ct +/− ) were intraperitoneally injected with zymosan, and PMN recruitment into the peritoneum at 2 h was assayed. ( b ) Time-course analyses of PMN accumulation at the peritoneum during zymosan-induced peritonitis. In addition to peritonitis, mice were induced colitis by 2% DSS. The SIRPα.ct −/− mice were characterized as having more severe DSS-induced colitis than their WT littermates, as determined by their lower survival rate ( c ) and more rapid weight loss ( d ). The data in a , b and d are presented as means±s.d., with n =6 in each condition. ( e ) In-vitro chemotaxis assay. PMN (2.5 × 10 6 ) obtained from SIRPα.ct −/− mice and WT littermates were induced by 10 μM fMLP to migrate across collagen-coated transwell filters. Transmigrated PMNs over a 1-h period were measured by an myeloperoxidase assay. The data are presented as means±s.d. and represent five independent experiments with triplicates per condition. ( f ) Reactive oxygen species production upon PMA challenge. PMN (5 × 10 5 ) from SIRPα.ct −/− mice and WT littermates were loaded with 200 μM luminol (Sigma). Following stimulation with PMA (1 μM), chemiluminescence was measured at 37 °C in relative light units (RLU) at every 30 s over a period of 30 min. ( g ) Illustration of co-adoptive transfer of PMNs from SIRPα.ct −/− and WT littermates followed by assay PMN infiltration during zymosan-induced peritonitis. ( h ) Infiltration of SIRPα.ct −/− PMN and SIRPα.ct +/+ PMN in the same WT mice at 2 h during zymosan–peritonitis. Note that SIRPα.ct −/− and WT PMNs were cross-labelled with either CFSE or DDAO-SE before transfer into the recipient mice. Fluorescence-activated cell sorting analyses of PMNs at 1 and 2 h ( i ) during peritonitis revealed more SIRPα.ct −/− PMN than WT PMN. ( j ) PMN phagocytosis of fluorescent beads coated with/without CD47 extracellular domain. SIRPα.ct −/− and WT PMNs were collected from the peritoneum during peritonitis at 3 h. ( k ) WT mice treated with water or DSS for 10 days were induced peritonitis by zymosan. PMNs collected from the peritoneum at 3 h were tested for phagocytosis. The results ( i , j and k ) are presented as means±s.d. with triplicates in each condition. * P <0.05; ** P <0.01 as assessed by Student’s t -test. Full size image Interestingly, in zymosan-induced peritonitis, we observed that the PMN numbers accumulating in the peritoneum at later time points (6 h) were lower in SIRPα.ct −/− mice compared with that in WT controls ( Fig. 5b ). As SIRPα-mediated signalling controls leukocyte phagocytosis [9] , [10] , we suspected that this PMN reduction in SIRPα.ct −/− mice at the later stage of peritonitis was due to enhanced phagocytic clearance. To test the PMNs’ phagocytic capability, PMNs isolated from the peritoneum during zymosan-induced peritonitis were incubated with fluorescent latex beads that were coated with or without a murine CD47 extracellular domain-Fc fusion protein. As shown in Fig. 5j , phagocytosis by SIRPα.ct −/− PMNs was significantly higher than that by SIRPα.ct +/+ PMNs from WT mice. Enhanced phagocytosis was also observed for the peritoneal PMNs isolated from mice that were treated with DSS for 10 days ( Fig. 5k ). Cleavage of SIRPα ITIMs by PMN serine proteases Analysis of the SIRPα gene determined that ITIM − SIRPα is not likely to be formed by conventional mRNA alternative splicing, as both ITIMs and the only translation termination codon are located in the same exon. Thus, one possible mechanism for generating ITIM − SIRPα in PMNs is that these cells possess specific enzymes that cleave the cytoplasmic tail of SIRPα at the post-translational level. To exclude the possibility that cleavage of SIRPα cytoplasmic ITIMs in PMNs is due to an enzymatic reaction during the cell lysis process, we directly fixed and permeabilized PMNs using cold alcohol (−20 °C, 20 min) and then labelled the cells with the anti-SIRPα.ct antibody. As shown in Fig. 6a , fluorescence-activated cell sorting analysis confirmed the cleavage of SIRPα cytoplasmic ITIMs in inflammatory PMNs but not in control PMNs from healthy donors. Interestingly, antibody labelling further indicated that C-terminally cleaved SIRPα is not uniform among PMNs in individual donors. 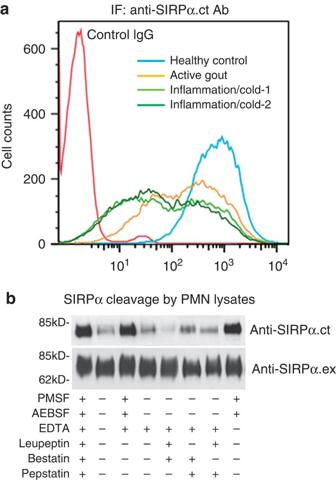Figure 6: Heterogeneous distribution of ITIM−SIRPα PMN and cleavage of SIRPα cytoplasmic ITIMs by PMN serine protease(s). (a) Fluorescence-activated cell sorting analysis of expression of SIRPα using anti-SIRPα.ct antibody in fixed and permeabilized PMN. PMN were isolated from one healthy donor, one donor with active gout (inflammatory arthritis) and two donors with throat and/or upper respiratory inflammation following a typical ‘cold’, respectively. (b) Cleavage of purified ITIM+SIRPα by PMN lysates and the effects of different protease inhibitors on SIRPα cleavage. The intact, ITIM+SIRPα was affinity purified from human monocytes using anti-SIRPα.ex-conjugated Sepharose.In-vitrocleavage reactions were performed by incubating aliquots of Sepharose-immobilized ITIM+SIRPα with 40 μl PMN lysates in the presence or absence of additional protease inhibitors, including phenylmethyl sulphonyl fluoride (PMSF; 3 mM), bestatin (50 μM), EDTA (10 mM), pepstatin (20 μM), leupeptin (200 μM) or AEBSF (10 mM). After the reaction, SIRPα was treated in SDS–PAGE sample buffer, followed by WB analysis. Figure 6: Heterogeneous distribution of ITIM − SIRPα PMN and cleavage of SIRPα cytoplasmic ITIMs by PMN serine protease(s). ( a ) Fluorescence-activated cell sorting analysis of expression of SIRPα using anti-SIRPα.ct antibody in fixed and permeabilized PMN. PMN were isolated from one healthy donor, one donor with active gout (inflammatory arthritis) and two donors with throat and/or upper respiratory inflammation following a typical ‘cold’, respectively. ( b ) Cleavage of purified ITIM + SIRPα by PMN lysates and the effects of different protease inhibitors on SIRPα cleavage. The intact, ITIM + SIRPα was affinity purified from human monocytes using anti-SIRPα.ex-conjugated Sepharose. In-vitro cleavage reactions were performed by incubating aliquots of Sepharose-immobilized ITIM + SIRPα with 40 μl PMN lysates in the presence or absence of additional protease inhibitors, including phenylmethyl sulphonyl fluoride (PMSF; 3 mM), bestatin (50 μM), EDTA (10 mM), pepstatin (20 μM), leupeptin (200 μM) or AEBSF (10 mM). After the reaction, SIRPα was treated in SDS–PAGE sample buffer, followed by WB analysis. Full size image To identify the possible enzyme(s) that are responsible for cleaving PMN SIRPα ITIMs, we purified homogeneous ITIM + SIRPα from human monocytes and performed in-vitro cleavage using PMN lysates prepared from the donors with inflammation (a PMN protease mixture) in the presence or absence of various protease inhibitors. As shown in Fig. 6b , the ITIM-containing cytoplasmic tail of SIRPα was cleaved after incubation with the PMN protease mixture. The cleavage of SIRPα ITIMs, however, was inhibited by the serine protease inhibitor phenylmethyl sulphonyl fluoride or AEBSF (4-(2-aminoethyl)benzenesulphonyl fluoride hydrochloride), but not by EDTA or other inhibitors. Thus, it is likely that certain leukocyte serine protease(s), but not metalloproteinases or other proteases, are responsible for the cleavage of SIRPα. We further identified the potential cleavage site on SIRPα. For this purpose, PMNs isolated from healthy donors and donors with inflammation were lysed by nitrogen cavitation and ultracentrifugation to prepare membrane-free cytosolic supernatant. The cleaved fragments of SIRPα in the supernatant were then immunoprecipitated using the anti-SIRPα.ct antibody. As shown in Supplementary Fig. S4 , two extra bands ( a and b , arrows) were obtained for the PMN supernatant prepared from the donors with inflammation compared with healthy controls. Whereas amino-terminal peptide sequencing yielded no results for band a , a six amino acid sequence, TSPQPA , was successfully produced from band b . The sequence matched that of the SIRPα cytoplasmic tail, suggesting that one of the SIRPα cleavage sites is likely at 461 Q–T 462 . ITIM-less SIRPα serves as a decoy receptor on PMNs Despite cleavage at the SIRPα cytoplasmic domain, the extracellular domain of SIRPα preserved binding to CD47. As shown in Fig. 7a , ITIM + SIRPα and ITIM − SIRPα proteins isolated from different PMN samples and PBMCs all directly and equally bound to CD47-AP ( Fig. 7b ) and CD47-expressing CHO cells [6] ( Fig. 7c ). In these binding assays, purified SIRPα proteins were immobilized in 96-well microtitre plates. After blocking, the wells were incubated with CD47-AP or CD47-expressing CHO cells in the presence or absence of inhibitory anti-CD47 or anti-SIRPα monoclonal antibodies ( Supplementary Fig. S4 ). These binding results strongly support that ITIM − SIRPα on PMNs likely serves as a decoy receptor that binds to CD47 but does not deliver inhibitory signalling. 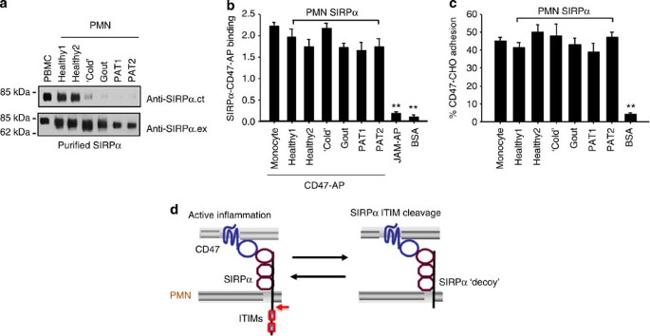Figure 7: The deletion of intracellular ITIMs does not affect the extracellular binding of SIRPα to CD47. Various SIRPα proteins, affinity purified from monocytes (PBMCs) and PMNs of healthy donors or donors under various inflammatory conditions, were confirmed as ITIM+SIRPα (from PBMCs or PMNs of healthy donors) or ITIM−SIRPα (from PMNs of inflammatory donors) by WB analyses (a). Purified SIRPα proteins were immobilized onto 96-well microtitre plates and then were incubated with 2 μg ml−1CD47-AP (b), or CD47-expressing CHO cells (CD47-CHO)6that were pre-loaded with BCECF (2',7'-bis-(2-carboxyethyl)-5-(and-6)-carboxyfluorescein) fluorescence dye (c). After washing, the binding of CD47-AP was assessed by measuring the AP activity. The paralleled binding of JAM-AP1, a chimera containing the extracellular domain of junctional adhesion molecule A (JAM-A), and BSA to immobilized SIRPα served as the non-binding controls. The adhesion of CD47-CHO cells to immobilized SIRPα was determined by measuring cell fluorescence intensity. CD47-CHO cell adhesion to BSA-coated wells served as a negative control. The results (means±s.d.) represent three independent experiments with triplicates in each condition. **P<0.01 assessed by Student’st-test. (d) Schematic illustration of the positive feedback loop mediated by inflammation-induced cleavage of SIRPα cytoplasmic ITIMs under chronic conditions. Figure 7: The deletion of intracellular ITIMs does not affect the extracellular binding of SIRPα to CD47. Various SIRPα proteins, affinity purified from monocytes (PBMCs) and PMNs of healthy donors or donors under various inflammatory conditions, were confirmed as ITIM + SIRPα (from PBMCs or PMNs of healthy donors) or ITIM − SIRPα (from PMNs of inflammatory donors) by WB analyses ( a ). Purified SIRPα proteins were immobilized onto 96-well microtitre plates and then were incubated with 2 μg ml −1 CD47-AP ( b ), or CD47-expressing CHO cells (CD47-CHO) [6] that were pre-loaded with BCECF (2',7'-bis-(2-carboxyethyl)-5-(and-6)-carboxyfluorescein) fluorescence dye ( c ). After washing, the binding of CD47-AP was assessed by measuring the AP activity. The paralleled binding of JAM-AP [1] , a chimera containing the extracellular domain of junctional adhesion molecule A (JAM-A), and BSA to immobilized SIRPα served as the non-binding controls. The adhesion of CD47-CHO cells to immobilized SIRPα was determined by measuring cell fluorescence intensity. CD47-CHO cell adhesion to BSA-coated wells served as a negative control. The results (means±s.d.) represent three independent experiments with triplicates in each condition. ** P <0.01 assessed by Student’s t -test. ( d ) Schematic illustration of the positive feedback loop mediated by inflammation-induced cleavage of SIRPα cytoplasmic ITIMs under chronic conditions. Full size image In this study we revealed an inflammation-induced structural and functional change in SIRPα in PMNs. Our results from PMNs obtained from human donors with various levels of inflammation and from two inflammatory mouse models clearly showed that the cleavage of the cytoplasmic ITIMs in PMN SIRPα was linked to various inflammatory conditions. Consistent with previous findings that SIRPα is a negative modulator of leukocyte inflammatory responses, our results further suggest that the inhibitory role of SIRPα relies on its cytoplasmic ITIMs and that the loss of these ITIMs can effectively remove the inhibition of PMN response by SIRPα. Given this dynamic interplay between PMN SIRPα and active inflammation, our results provide a novel SIRPα-based positive feedback loop in inflammatory regulation. As depicted in Fig. 7d , inflammation induces the specific cleavage of signalling SIRPα ITIMs without affecting extracellular CD47-SIRPα binding, leading to the formation of a SIRPα ‘decoy’ and an enhancement of PMN inflammatory response. The conversion of a signalling SIRPα to a non-signalling ‘decoy’ receptor by active inflammation is in fact not an isolated case in the immunological regulatory system. Several important cell surface receptors, including receptors for inflammatory cytokines (for example, IL-1 and IL-13), have been found to be expressed as both signalling receptors and non-signalling ‘decoys’ under various conditions [26] , [27] , [28] . Previous studies showed that PMNs express receptors for a range of inflammatory cytokines [29] , indicating that these cells are subject to inflammatory regulation. Although the trigger molecule(s) that initiate PMN SIRPα cleavage have not been determined, several pieces of evidence suggest the involvement of certain proinflammatory cytokines or factors that are induced during the ‘post-acute’ phase of active inflammation, as the loss of PMN SIRPα ITIMs occurs at this stage. Studying DSS-induced colitis, we found that serum IL-17 levels were significantly elevated at the ‘post-acute’ stage and that the kinetics of IL-17 levels correlated with SIRPα ITIM cleavage in PMNs ( Fig. 3 ). The neutralization of serum IL-17 by an anti-IL-17 antibody effectively blocked the cleavage of SIRPα ITIMs in PMNs ( Fig. 4 ). In contrast, the direct treatment of healthy control mice with IL-17 elicited the cleavage of PMN SIRPα ITIMs ( Fig. 4 ). In fact, among the cytokines that we tested, including IL-17, tumour-necrosis factor-α, interferon-γ, IL-1, IL-6, IL-10 and IL-13, IL-17 was the only cytokine that highly increased in the sera of DSS-treated mice, especially at the ‘post-acute’ stage. It is clear that IL-17 acts as a proinflammatory cytokine that is tightly associated with the promotion of inflammation at the ‘post-acute’ stage. Here we provide evidence that IL-17 directly potentiates the PMN response by partly inducing the cleavage of SIRPα ITIMs. Such a change in PMN SIRPα results in enhanced PMN chemotaxis, reactive oxygen species release and phagocytosis. In addition to IL-17, we also tested other known PMN-priming factors, such as lipopolysaccharides, N-formyl- L -methionyl- L -leucyl-phenylalanine (fMLP) and chemokine (C-X-C motif) ligand 1 (CXCL1), for the ability to induce SIRPα ITIM cleavage. By treating mice with lipopolysaccharides, fMLP or chemokine (C-X-C motif) ligand 1 (CXCL1), we found that each treatment produced truncated SIRPα, albeit to various degrees ( Supplementary Fig. S5 ), suggesting that the priming of PMNs by these factors is also associated with SIRPα ITIM cleavage. In summary, our findings of PMN SIRPα cleavage and enhanced PMN recruitment along with an elevation of proinflammatory cytokines indicate that PMNs are dynamically regulated at different stages of active inflammation. It is worth noting that SIRPα.ct −/− mutant mice are associated with defective dendritic cell (DC) maturation and function [24] , [30] , [31] . As a result, SIRPα.ct −/− mice have an inadequate differentiation of CD4 + T cells into Th cells. This defective DC-induced T-cell function explains the resistance of the mice to disease conditions that are dependent on elevated Th1 or Th17 functions [24] , [32] , [33] . Previous studies also demonstrated that IL-10 −/− mice backcrossed with SIRPα.ct −/− mice were protected from spontaneous colitis [33] . The specific case of colitis occurring in IL-10 −/− mice is essentially a consequence of mucosal intolerance to luminal antigens, in which DC-mediated antigen presentation, which induces proinflammatory Th cells, have a crucial role [34] , [35] . As SIRPα mutation causes defective DC function, resulting in a lack of induction of activating Th cells, it is comprehensible that a SIRPα.ct −/− phenotype provides resistance to spontaneous colitis in IL-10 −/− mice [33] . Although SIRPα.ct −/− mice do not spontaneously develop colitis, acute colitis can be induced in these mice by DSS treatment. In this colitis, macrophages and PMNs control the early phase of pathogenesis (<6 days of DSS treatment), whereas DCs and T cells mainly contribute to the ‘post-acute’ and chronic phases (>day 7) [20] , [21] . In the current study we found that SIRPα.ct −/− mice displayed a substantially enhanced inflammatory condition at the early stage during the DSS treatment, and this severe colitis, primary due to enhanced PMN (also macrophage) responses, result in animal annihilation before the condition proceeding to the chronic phase. Our results suggest that the loss of SIRPα cytoplasmic ITIMs is due to inflammation-induced enzymatic cleavage. Although the responsible enzyme(s) are not identified at this stage, several PMN-specific serine proteases might be involved in cleaving SIRPα cytoplasmic ITIMs and enhancing PMN inflammatory responses. In support of this phenomenon, the activities of serine proteases in PMNs were found to be increased after stimulation with various inflammatory factors [36] , [37] . In addition, PMN serine proteases are well known for their ability to modulate many important molecules in PMNs, including CD11b (ref. 38 ) and IL-18 (ref. 39 ). In agreement with our finding that SIRPα ITIMs are cleaved in PMNs but not in monocytes under inflammatory conditions, these serine proteases are enriched in PMNs but not in monocytes. In summary, we identified a novel SIRPα-based positive feedback loop under various chronic inflammatory conditions. When an inflammatory condition prolongs, elevated inflammatory factors, such as IL-17, can prime PMNs to a highly responsive state by removing the inhibitory signalling effects by SIRPα. Thus, this study provides new insight into inflammatory diseases and will aid the future design of novel anti-inflammatory therapeutic strategies. Antibodies A polyclonal antibody against the SIRPα extracellular domain, anti-SIRPα.ex, was generated by immunization of rabbits with SIRPα.ex-glutathione S -transferase (GST), a recombinant fusion protein containing the entire SIRPα extracellular domain [1] . IgG was purified from serum, and its cross-reactivity with the SIRPβ extracellular domain was minimized by passage through SIRPβ.ex-GST-conjugated Sepharose. As shown in Supplementary Fig. S1 , this anti-SIRPα.ex antibody does not cross-react with SIRPβ. Mouse polyclonal antibodies against the SIRPα extracellular IgV loop (anti-IgV) and the IgC loops (anti-IgC), and antibodies targeted against different regions of the SIRPα intracellular domain (YT-1, amino acids 457–504; YT-2, amino acids 433–504; and YT-3, amino acids 398–504) were generated by immunizing BALB/c mice with the recombinant proteins SIRPα.IgV-Fc, SIRPα.IgCs-Fc, YT-1-GST, YT-2-GST and YT-3-GST, respectively. A rabbit polyclonal antibody that specifically detects the SIRPα intracellular C-terminus, anti-SIRPα.ct, was raised using the synthetic peptide PKPEPSFSEYASVQVPRK, corresponding to the C-terminus of SIRPα. A rat anti-mouse SIRPα extracellular domain monoclonal antibody (clone P84), an anti-SIRPβ antibody (clone B4B6) and antibodies detecting mouse IL-17 and IL-6 were purchased from BD Biosciences (San Jose, CA). A low-endotoxin, azide-free anti-mouse IL-17A antibody was purchased from BioLegend (San Diego, CA). Animals Adult, female mice (6- to 10-week-old, 20–22 g) in C57BL/6J background were used in the study. SIRPα.ct −/− mice (also termed as SHP substrate-1 mutant mice) that express a mutant form of SIRPα, which lacks most of the cytoplasmic region [24] , were backcrossed onto the C57BL/6J background for ten generations. The mice were bred and maintained at the Animal Facility of Georgia State University under pathogen-free conditions. All experiments using animals and procedures of animal care and handling were performed following protocols approved by the Institutional Animal Care and Use Committee of Georgia State University (Atlanta, GA). Construction of the recombinant fusion proteins The entire SIRPα.ex was amplified by PCR from the Marathon-ready complementary DNA libraries of human leukocytes (Clontech) using the primers SP1 (5′-cagaagcttccgcggcccatggagcccgcc-3′) and SP2 (5′-ttgattagatctagtgttctcagcggcggtatt-3′). The amplified DNA fragment was cloned into a pcDNA3.1 vector that had been preconstructed with GST (a gift from Dr A Ullrich). The plasmid containing the membrane-distal IgV loop, Ig loop (2+3) and Ig loop 3 of SIRPα and rabbit Fc (SIRPα.IgV-Fc) fusion was generated previously [6] , [40] . To generate recombinant GST fusion proteins containing various regions of the SIRPα intracellular domain, PCRs were performed with the sense primer YT-1 (5′-ataggatcccagaccagcccgcagcccgc-3′), YT-2 (5′-ataggatccaacctgcccaaggggaagaa-3′) or YT-3 (5′-ataggatcccagaagaaagcccagggctc-3′) paired with the antisense primer cSIRPα.xho (5′-ttgctcgagtcacttcctcgggacctggac-3′). The amplified DNA fragments were cloned into the pGEX4.1 vector through the Bam HI and Xho I sites. GST fusion proteins were produced in BL21 bacteria with 1 mM isopropylthiogalactoside induction, followed by affinity purification using glutathione–Sepharose. These fusion proteins were used to immunize mice to obtain the polyclonal antibodies YT-1, YT-2 and YT-3. PMN and PBMC isolation The use and handling of human blood samples in this study was approved by the institutional review boards of Nanjing University (Nanjing, China) and Georgia State University, and written informed consent was obtained from each participant. Leukocytes were isolated from the whole blood of human volunteers or mice as previously described [41] . Briefly, fresh heparinized blood from healthy human volunteers was subjected to dextran sedimentation followed by Ficoll-Hypaque gradient centrifugation. Contaminating red blood cells were removed by NH 4 Cl lysis. PMNs were counted using a Coulter ZM counter, resuspended in HEPES-buffered RPMI 1640 medium at 10 7 cells per ml and maintained on ice until use. To inhibit proteolysis during cell lysis, the cells were pretreated with 2.5 mM diisopropylfluorophosphate for 30 min at room temperature. The activation status and chemotactic efficacy of the isolated PMNs were examined using a rapid assay [42] . To obtain mouse bone marrow cells, femur bone cavities were opened by cutting off both ends of the bone, and bone marrow cells were flushed out using Hank’s buffer devoid of Ca 2+ and Mg 2+ , followed by the lysis of red blood cells. In certain experiments, the bone marrow leukocytes were further separated to obtain a population of mature PMNs. Western blot detection of protein expression Freshly isolated PMNs and PBMCs (5 × 10 7 each) were lysed in lysis buffer containing 100 mM Tris (pH 7.5), 1% Triton X-100, a 1:100 dilution of a protease inhibitor cocktail and 3 mM phenylmethyl sulphonyl fluoride (Sigma). The cell lysates were subject to SDS–PAGE and western blot (WB) analyses using the antibodies (2 μg ml −1 monoclonal antibody, 1:200–2,000 dilution of polyclonal antibody) against the different regions of the SIRPα protein, including the anti-SIRPα.ex and anti-SIRPα.ct antibodies. For protein deglycosylation, 100 μl cell lysate was denatured, reduced and digested with 100 units of PNGase F (New England Biolabs, Ipswich, MA) in the presence of 1% NP-40 at 37 °C. Uncut, original images of important WB were provided in Supplementary Figs S6–S9 . PMN transmigration assays An in-vitro PMN transmigration assay using collagen-coated, permeable transwell filters (0.33 cm [2] , 5 μm pore size) has been previously established [42] . Briefly, murine PMNs in 150 μl Hank’s Balanced Salt Solution were added to the upper transwell chambers of 24-well plates, and transmigration was initiated by adding 10 μM fMLP in 0.5 ml Hank’s Balanced Salt Solution to the lower chambers, followed by incubation at 37 °C. PMNs that transmigrated to the lower chambers at different times were measured by a myeloperoxidase assay. A zymosan-induced murine acute peritonitis model was used to assay PMN infiltration in vivo . For these experiments, mice (20–22 g) were injected intraperitoneally with 0.5 mg zymosan A (Sigma) prepared in 0.5 ml sterile saline, followed by euthanasia after various time periods. The peritoneal cavities were then lavaged with 3 ml cold PBS containing 2 mM EDTA. PMNs that infiltrated into the peritoneum were collected and analysed by myeloperoxidase assay or immunofluorescence labelling using a PE-conjugated anti-Ly6G antibody (eBioscience, San Diego, CA). Adoptive transfer assay of PMN infiltration For these experiments, isolated bone marrow cells from SIRPα.ct −/− mice and their WT littermates were labelled with CFSE and DDAO-SE (both from Invitrogen). The same numbers of labelled bone marrow PMNs from SIRPα.ct −/− and WT mice were transferred into healthy recipient mice. Peritonitis was then induced using zymosan in the recipient mice to test the infiltration of labelled PMNs into the peritoneum. Labelled PMNs in the peritoneal lavage were assayed by flow cytometry or examined by fluorescence microscopy. Inflammatory mouse models DSS-induced colitis [18] and STZ-induced hyperglycaemia [19] were established in C57BL/6J mice. To induce colitis, 2% DSS (MP Biomedicals, Santa Ana, CA) prepared in pure water was given to the mice as their drinking water. The mice were inspected daily for distress and colitis symptoms. To induce hyperglycaemia, C57BL/6J mice were fasted for 4 h, followed by an intraperitoneal injection with STZ (Sigma) at a dose of 50 mg kg −1 body weight for 5 consecutive days. The blood glucose levels of the mice were tested 6 days after the injections to confirm hyperglycaemia, and the mice were used in a study of SIRPα expression and PMN function 2–3 weeks after the hyperglycaemic condition was established. Phagocytosis assay Fluorescent latex beads (1.0 μm in diameter; Polyscience Inc., Warrington, PA) were coated with or without 1 mg ml −1 recombinant murine CD47-Fc. The beads were opsonized with the subject’s serum for 30 min at 37 °C and then washed with PBS and adjusted to 2.5 × 10 7 /50 μl in PBS. Peritoneal PMNs were isolated from water- or DSS-treated mice at 4 h post injection with zymosan A. PMN were then incubated with fluorescent beads (25 μl each) at 37 °C for 30 min. The incubation was stopped by placing the samples on ice, and the samples were washed twice with PBS. Flow cytometric analyses were performed to assay the phagocytic capacity of the PMNs. Purification of SIRPα Intact ITIM + SIRPα or ITIM − SIRPα was purified from monocytes or inflammatory PMNs using an anti-SIRPα.ex antibody affinity column. The anti-SIRPα.ex antibody was conjugated to cyanogen bromide-activated Sepharose 4B (2 mg protein per ml Sepharose). Freshly isolated human PMNs and PBMCs were lysed in the presence of protease inhibitors, followed by incubation with anti-SIRPα.ex-conjugated Sepharose for 4 h (4 °C). The Sepharose–protein complexes were then washed using a buffer containing 1% octylglucoside, followed by the elution of SIRPα with 100 mM acetate buffer (pH 4) containing 100 mM NaCl and 1% octylglucoside. Purification of cleaved SIRPα fragment and N-terminal sequencing Freshly isolated PMN (1 × 10 8 ) from healthy controls and patients were suspended in 3 ml of nitrogen cavitation buffer (0.34 M sucrose, 10 mM HEPES, 1 mM EDTA, 0.1 mM MgCl 2 , 1 mM Na 2 ATP, pH 7.4) followed by nitrogen cavitation lysis (15 min, 400 p.s.i., 4 °C). After ultracentrifugation (170,000 g ; 3 h, 4 °C), the supernatants were subjected to immuneprecipitation by anti-SIRPα.ct antibody-conjugated Sepharose. After extensive washing, the beads were boiled in sample buffer and proteins were separated by SDS–PAGE using a 20% polyacrylamide gel followed by staining with Gelcode blue (Pierce). The cleaved SIRPα bands that were confirmed by WB analyses were excised for N-terminal amino acid sequencing. How to cite this article: Zen, K. et al. Inflammation-induced proteolytic processing of the SIRPα cytoplasmic ITIM in neutrophils propagates a proinflammatory state. Nat. Commun. 4:2436 doi: 10.1038/ncomms3436 (2013).